A general ligand design for gold catalysis allowing ligand-directed anti-nucleophilic attack of alkynes Most homogenous gold catalyses demand ≥0.5 mol% catalyst loading. Owing to the high cost of gold, these reactions are unlikely to be applicable in medium- or large-scale applications. Here we disclose a novel ligand design based on the privileged (1,1′-biphenyl)-2-ylphosphine framework that offers a potentially general approach to dramatically lowering catalyst loading. In this design, an amide group at the 3′-position of the ligand framework directs and promotes nucleophilic attack at the ligand gold complex-activated alkyne, which is unprecedented in homogenous gold catalysis considering the spatial challenge of using ligand to reach anti-approaching nucleophile in a linear P-Au-alkyne centroid structure. With such a ligand, the gold(I) complex becomes highly efficient in catalysing acid addition to alkynes, with a turnover number up to 99,000. Density functional theory calculations support the role of the amide moiety in directing the attack of carboxylic acid via hydrogen bonding. One of the exciting thrusts in organic synthesis in the past dozen years is homogenous gold catalysis [1] , [2] , [3] , [4] , [5] , [6] , [7] . Various versatile synthetic methods, offering efficient access to a broad array of functional structures, have been developed based on an initial coordination of a C-C triple bond to an LAu + , a cationic gold(I) species with one coordinating ligand (that is, L) and a subsequent anti-attack by a nucleophile at the alkyne ( Fig. 1a ). Owing to the linear nature of the L-Au-alkyne complex and, making the matter worse, to the anti-nucleophilic approach, it is highly challenging to introduce bonding interaction between the ligand and the nucleophile due to apparent spatial constrain. To date, there is no reported reaction of this nature. Although in enantioselective gold catalysis [8] , [9] , ligands/counter anions to the metal centre could impose a chiral environment in the approaching path of nucleophiles (often with allene substrates), the controls are invariably steric and offer little, if not to the opposite effect, rate acceleration or efficiency improvement. 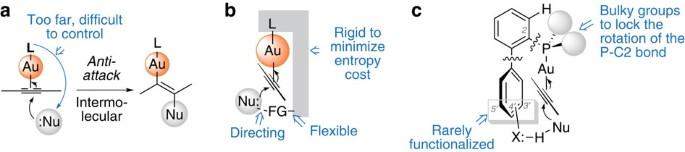Figure 1: A novel ligand design for highly efficient gold catalysis. (a)Anti-attack at gold(I)-activated alkyne by a nucleophile. (b) A general concept to achieve quasi-intramolecular, ligand-directed nucleophilic attack. (c) A design based on (1,1′-biphenyl)-2-ylphosphine framework. Figure 1: A novel ligand design for highly efficient gold catalysis. ( a ) Anti -attack at gold(I)-activated alkyne by a nucleophile. ( b ) A general concept to achieve quasi-intramolecular, ligand-directed nucleophilic attack. ( c ) A design based on (1,1′-biphenyl)-2-ylphosphine framework. Full size image On the other hand, with a few exceptions [10] , [11] , [12] , [13] , [14] , [15] , most homogenous gold catalyses demand ≥0.5 mol% catalyst loading. Because of the high cost of gold, these reactions are unlikely applicable in medium- or large-scale applications, which in turn has continuously reinforced the prevailing perception that gold chemistry would be too expensive to be useful for industrial scale processes. This general shortcoming in gold catalysis could be overcome by substantially improving the turnover numbers (TONs) of gold catalysts and hence dramatically lowering their loadings. Ligand design [16] is a well-practiced strategy in transition metal catalysis to achieve high catalyst TONs, but little success [14] , [15] has been reported in this regard in homogenous gold catalysis. Herein we disclose a ligand design that offers a conceptually new and potentially general approach to achieving highly efficient gold catalysis with ultra-low catalyst loadings. With an optimized ligand based on the privileged (1,1′-biphenyl)-2-ylphosphine framework, yet possessing an unprecedented and strategical 3′-amide group, additions of a diverse range of carboxylic acids to alkynes are achieved with typically p.p.m.-level catalyst loadings and catalyst TON up to 99,000. Design and synthesis of novel biarylphosphine ligands It is envisioned that a ligand with a rigid and extending framework could project a functional group (FG) farther enough to reach to an approach nucleophile ( Fig. 1b ) [17] . The FG could be designed such that it could have attractive interaction with the nucleophile and hence be capable of directing its attack at the gold-activated triple bond. The rigidity of the backbone would minimize the entropy cost for organizing transition states, and the directing group should be flexible enough to accommodate a broad substrate scope. This strategy is expected to facilitate the initial nucleophilic attack drastically by converting it from an intermolecular process to a quasi-intramolecular event and may also accelerate subsequent transformations. As a result, higher catalyst TONs and hence more efficient catalysis could be expected. Herein we report an implementation of this design in a gold-catalysed addition of carboxylic acids to alkynes with catalyst TONs up to 99,000, a broad reaction scope and high-to-excellent efficiencies; moreover, the general applicability of the design in other gold catalyses is demonstrated by highly efficient hydration and hydroamination of alkynes. Bulky and electron-rich biarylphosphines developed by Buchwald [18] , [19] , [20] belong to a privileged class of phosphorus-based ligands that are versatile for promoting various Pd catalysis [21] , [22] . Lately, these ligands have been borrowed in gold catalysis with much success [23] , [24] , [25] , [26] , [27] , [28] , [29] , [30] , but modification of them for gold catalysis is rare [31] . Perhaps, owing to the nature of Pd catalysis, the lower half of the bottom phenyl ring of these ligands (that is, C3′, C4′ and C5′) has seldom been substituted with FGs. The only exceptions are a 3′-sulphonate derived from SPhos and a 4′-sulphonate from XPhos for the purpose of increasing catalyst aqueous solubility [32] . In contrast to square planar Pd(II) complexes, bis-coordinated gold(I) complexes exhibit linear structures, which should invite a ligand design philosophy different from that for Pd catalysis. In the context of the biarylphosphine ligands ( Fig. 1c ), by fixing the P-C2 rotation using bulky substituents on the phosphorus, the linear P-Au-alkyne axis should be parallel to and bisect the pendant phenyl ring, thus putting the coordinated alkyne alongside the lower half of that ring. It is envisioned that if these remote positions on that part of the phenyl ring, with the activated alkyne closely positioned, were to be functionalized with H-bond acceptors, these FGs could extend further enough to direct neutral nucleophiles via H-bonding interactions and/or proton stabilization to attack the activated alkyne in an ‘intramolecular’ anti-attack. In this manner, the design concept shown in Fig. 1b could be implemented. To put this concept into practice, we designed a series of (1,1′-biphenyl)-2-yldi(adamantan-1-yl)phosphine ligands (that is, L1 – L8 ) with either C3′ or C4′ functionalized ( Table 1 ). They can be readily synthesized via consecutive cross-couplings of 1,2-dihalobenzene with arylboronic acids and di(adamantan-1-yl)phosphine (Ad 2 PH). Ad 2 P was chosen because of its ease of installation [33] and, more importantly, the steric bulk of the Ad groups. The structure of the ligand L8 is confirmed by the X-ray diffraction study of its gold complex L8AuCl ( Fig. 2 ). Table 1 New ligands prepared in study and C=O stretching wavelengths of carbonyls in ligands and catalysts. 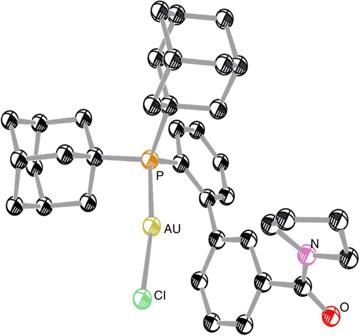Figure 2: The ORTEP drawing ofL8AuClat 50% ellipsoid probability. For details seeSupplementary Table 1. Full size table Figure 2: The ORTEP drawing of L8AuCl at 50% ellipsoid probability. For details see Supplementary Table 1 . Full size image Screening ligands to maximize catalyst TONs The addition of a carboxylic acid to an alkyne is chosen as the model reaction. This transformation has been previously realized using 5 mol% Ph 3 PAuCl/AgPF 6 with catalyst TONs up to 18 (ref. 34 ), and the best catalyst TON (that is, 124) of this type of reaction was achieved via Ru catalysis [35] . Importantly, the alkenyl ester products possess mildly activated acyl groups and are versatile substrates of broad synthetic utilities. As shown in Table 2 , with IPrAuNTf 2 , a catalyst only different by the counter anion from the previously reported p.p.m.-level IPrAuCl/AgSbF 6 for alkyne hydration in 1,4-dioxane/H 2 O (ref. 12 ), there was only trace amount of the desired 2-dodecenyl benzoate (that is, 1a ) detected under the indicated conditions (entry 1). While a basic dimethylamino group at the 4′-position in the case of the ligand L2 did not offer any improvement (entry 3), its regioisomer L1 with the substituent at the 3′-position led to some notably improvement (entry 2), hinting that substitution at C3′ might be better than at C4′ for the reaction. With piperidin-1-ylcarbonyl as the FG at either the 4′- or the 3′-position in the case of ligand L3 or L7 , respectively, a much more efficient reaction with an observed catalyst TON of 80 was realized, suggesting that an amide is a suitable FG for promoting the reaction (entries 4 and 5). By lowering down the gold loading to 0.11%, the TONs reached 609 for L3 (entry 6) and 827 for L7 (entry 7), which are much better than the Ru case [35] , and was further increased to 1,681 (entry 8) by further decreasing the loading of the better gold complex L7AuCl . With little success with other FGs at the 3′-position, the reaction optimization was then focused on modifying the amide group of L7 , and the results are shown in entries 9–12. Whereas L8 with a 3′-(pyrrolidin-1-ylcarbonyl) group turned out to be the most efficacious ligand, a qualitative inverse correlation between the reaction yields and the wavenumbers of the amide carbonyl stretching band ( ν C=O ) of both the ligands and the corresponding gold complexes is revealed. The higher the ν C=O , the less basic the carbonyl oxygen is and hence the weaker H-bond acceptor. Therefore, the reaction yield positively correlates to the H-bond acceptor capacity of the amide carbonyl oxygen. This qualitative trend is consistent with the design that necessitates the remote FG to recruit the nucleophile via H-bonding. After further optimization, the catalyst TON using the best ligand L8 could reach 34,400 in 12 h with 25 p.p.m. of its cationic gold complex in fluorobenzene when NaBARF (sodium tetrakis[3,5-bis(trifluoromethyl)phenyl]borate, 0.12%) was added (entry 14), while a 40-p.p.m. catalyst loading allowed full conversion under the same conditions (entry 13). The role of NaBARF is probably to prevent catalyst deactivation by scavenging coordinating anionic impurities. In comparison, under the same conditions a catalyst TON of 40 was reached for JohnPhosAuNTf 2 (entry 15). By considering that t -butyl and 1-adamantyl have similar steric bulk, the rate acceleration of 860-fold by L8AuNTf 2 over JohnPhosAuNTf 2 can be attributed to the mere incorporation of the remote 3′-amide group. Table 2 Screening various ligands and the optimization of reaction conditions. Full size table The reaction scope with ultra-low catalyst loadings With the low submicromolar catalysis realized, its applicability to other carboxylic acids was first examined using 1-hexyne or 1-dodecyne as the alkyne partner. As shown in Fig. 3a , various acids possessing a diverse range of FGs were allowed, mostly resulting in near quantitative yields while with a catalyst loading of 100 p.p.m. or less. Some notable FGs include Bpin (for example, 1h ), thiophene (for example, 1i ), diene (for example, 1l ), different halogens (for example, 1e - 1g , 1p and 1q ) and protected α-amino groups (for example, 1t and 1u ). Whereas the reaction of N -protected proline leading to 1t require higher catalyst loading, the reaction of much more acidic trifluoroacetic acid was realized with 10 p.p.m. catalyst, giving a catalyst TON of at least 99,000. In addition, hindered acids such as 1-adamentanecarboxylic acid (in the case of 1n ) and 2,6-dichlorobenzoic acid (in the case of 1g ) reacted smoothly. The scope with different alkynes was then probed using benzoic acid. As shown in Fig. 3b , terminal alkynes with different functionalities and internal alkynes were all suitable substrates, and the reaction yields were mostly nearly quantitative. These reactions, however, generally required higher catalyst loadings. In the cases of an enyne (that is, 1z ) and non-activated internal alkynes (that is, 1aa and 1ab ), the catalyst loadings were relatively high, probably because of lower reactivities of these substrates in comparison with aliphatic terminal alkynes. 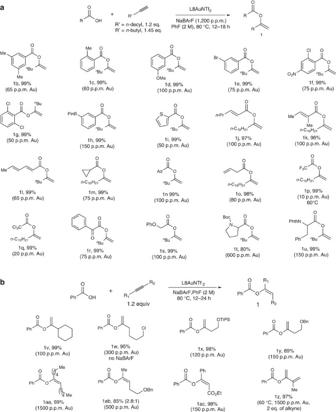Figure 3: The reaction scope with isolated yields reported. (a) Reactions of various acids with 1-hexyne or 1-dodecyne. (b) Reactions of various alkynes with benzoic acid. Reactions run under N2in vial. NaBARF, sodium tetrakis[3,5-bis(trifluoromethyl)phenyl]borate. Figure 3: The reaction scope with isolated yields reported. ( a ) Reactions of various acids with 1-hexyne or 1-dodecyne. ( b ) Reactions of various alkynes with benzoic acid. Reactions run under N 2 in vial. NaBARF, sodium tetrakis[3,5-bis(trifluoromethyl)phenyl]borate. Full size image This dramatic increase of catalyst TON in this gold catalysis using the remotely amide-functionalized L8 as a ligand can be ascribed to the H-bonding between the ligand amide group and the approaching carboxylic acid, which makes the reaction quasi-intramolecular and hence decrease of the entropy loss in the transition state; moreover, it materializes a general base catalysis by the basic amide moiety through which the nucleophilicity of the acid is enhanced. In addition, the protonated amide after the initial step should serve as intramolecular proton source for rapid protodeauration and hence accelerate catalyst turnover. To substantiate this rationale and, hence, to offer theoretical support to our design, density functional theory (DFT) [36] , [37] studies were performed with GAUSSIAN09 (ref. 38 ) program and PBE1PBE [39] , [40] method. In the calculation, the ligand L8 , one molecule of benzoic acid and one molecule of propyne were used; moreover, 6–31+G** basis set was used for the reactants, the NTf 2 − anion and the 3′-(pyrrolidin-l-ylcarbonyl) group, 6-311+G** basis set was used for P, 6-31G* basis set was used for other atoms in the ligand and the SDD basis set with an effective core potential [41] was used for Au. Geometry optimization was performed in dichloroethane using the SMD [42] method. Harmonic vibration frequency calculations were carried out and each of the optimized transition states has one imaginary frequency. We proposed that, in the catalytic reaction with JohnPhos as the ligand, the NTf 2 − counter anion will activate the benzoic acid and assist the proton transfer process [43] , [44] , [45] . However, in the catalytic reaction with L8 , the amide group is a better alternative to the NTf 2 − anion. To facilitate the comparison of these two scenarios, a reaction pathway using L8 as the ligand but without involving its 3′-amide group was used to mimic the case of JohnPhos. As shown in Fig. 4 , in the transition state TS- NTf 2 , the NTf 2 − anion stabilize the proton of the benzoic acid while its carbonyl oxygen attacks the C2 of propyne; notably, the amide group is a bystander. In TS- Amide , the amide group stabilizes the proton, and the NTf 2 − anion is far away from the reaction centre, binding to the system via weak hydrogen bonds. The TS- Amide is 2.1 kcal mol −1 more favourable in free energy than TS- NTf 2 , consistent with the experimental observation that L8 is a better ligand than JohnPhos. In addition, in TS- Amide NTf 2 − does not participate in the reaction and hence needs not to be bound [45] . Such a binding in TS- Amide causes rigid body translational and rotational entropy loss, which was estimated to be 3.6~4.8 kcal mol −1 for the binding of small molecules to protein [46] . On the basis of this estimation, TS- Amide should be more than 5 kcal mol −1 more favourable than TS- NTf 2 , which is in line with the observed 860-fold increase of the TONs as the estimated energy barrier difference is around 4.7 kcal mol −1 if the TON difference is treated as the rate difference. These theoretical studies corroborate that the basic amide group and the intramolecular nature of the reaction are critical for the much enhanced TONs. 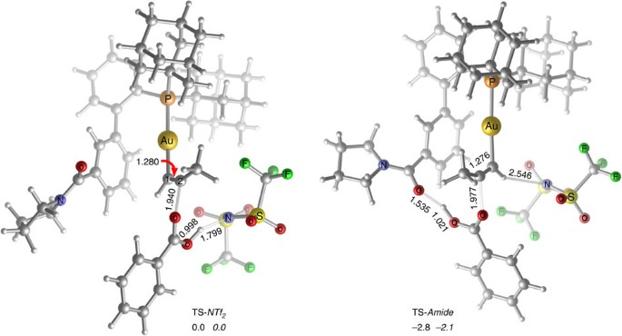Figure 4: Optimized transition states. The optimized NTf2−anion activated transition stateTS-NTf2and amide group activated transition stateTS-Amide. The selected bond lengths are in angstroms, the relative energies ΔEsoland free energies ΔGsol(in italic, 298 K) in dichloroethane are in kcal mol−1. Figure 4: Optimized transition states. The optimized NTf 2 − anion activated transition state TS- NTf 2 and amide group activated transition state TS- Amide . The selected bond lengths are in angstroms, the relative energies Δ E sol and free energies Δ G sol (in italic, 298 K) in dichloroethane are in kcal mol −1 . Full size image The remote amide group in L8 can also facilitate nucleophilic attack by H 2 O, resulting in substantially accelerated hydration of alkynes. As shown in Table 3 , when the reaction was run in non-polar toluene with two equivalents of H 2 O, L8 was a much more effective ligand than the remotely non-functionalized 2-biphenyphosphine ligand JohnPhos and the NHC ligand IPr; the same trend was observed with methanol as solvent, and notably without optimization the hydration was easily accomplished with 100 p.p.m. of L8AuNTf 2 and a catalyst TON of at least 10,000. These results again highlight the essential role of the remote amide group, and more importantly suggest that the design principle can be generally applicable to other reactions. To further substantiate the point, we performed hydroamination of alkynes with aniline. As shown in Fig. 5a , using L8AuNTf 2 as the catalyst, its TONs with phenylacetylene as the substrate reached 8,500, a nevertheless pleasing number albeit lower than 22,000 achieved by the catalyst developed by Lavallo [14] ; however, with 1-dodecyne as the substrate, L8AuNTf 2 was a much better catalyst than that by Lavallo as its TON reached 3,900 while a TON of 435 is reported in the latter case. Table 3 Gold-catalyzed alkyne hydration. 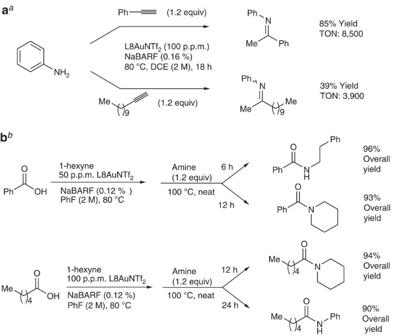Figure 5: Synthesis of imines and amides. (a) Gold-catalysed hydroamination of alkynes. (b)Application in amide synthesis.aNMR yields using diethyl phthalate as the internal reference.bIsolated yields. DCE, 1,2-dichloroethane; NaBARF, sodium tetrakis[3,5-bis(trifluoromethyl)phenyl]borate. Full size table Figure 5: Synthesis of imines and amides. ( a ) Gold-catalysed hydroamination of alkynes. ( b )Application in amide synthesis. a NMR yields using diethyl phthalate as the internal reference. b Isolated yields. DCE, 1,2-dichloroethane; NaBARF, sodium tetrakis[3,5-bis(trifluoromethyl)phenyl]borate. Full size image The utility of this chemistry is exemplified by a two-step, high yielding synthesis of amides ( Fig. 5b ), where the gold catalysis offered mild activation of carboxylic acids in a highly efficient manner. A notable advantage of this amide formation is that the by-product is 2-hexanone, which is volatile and can be readily removed under vacuum. In summary, we have advanced a novel ligand design based on the privileged (1,1′-biphenyl)-2-ylphosphine framework that could dramatically improve gold catalysis. It employs FGs at the remote 3′-position to direct and promote nucleophilic attack of gold-activated alkynes, which is unprecedented in homogenous gold catalysis considering the spatial challenge of using ligand to reach anti-approaching nucleophile in a linear L-Au-alkyne centroid structure. With a basic, H-bond accepting (pyrrolidin-1-yl)carbonyl group at the 3′-position, the gold(I) complex derived from the biarylphosphine ligand becomes highly efficient in catalysing acid addition to alkynes, with its TON up to 99,000. DFT calculations support the role of the amide moiety in directing the attack of carboxylic acid via H-bonding. Further applications of this catalyst to hydration and hydroamination of alkynes similarly realized high catalyst TONs, therefore confirming the general applicability of this ligand design. We anticipated that this design and the general principle of engaging bonding interactions between ligand and reactants could be employed to substantially improve an array of other gold catalyses, thereby promoting the application of gold chemistry in industrial scale processes, and might also be useful for improving catalysis by other transition metals. General procedure for synthesis of ligand and catalyst As shown in Fig. 6 , to a dispersion of 10 mmol 3-iodobenzoic acid (1 equiv) in 50 ml dry CH 2 Cl 2 was added 25 mmol oxalyl chloride (2.5 equiv) and three drops of N , N -dimethylformamide (DMF), and the mixture was stirred for 2–4 h at room temperature. The reaction mixture was evaporated under reduced pressure and dried under vacuum to yield 3-iodobenzoyl chloride, which was dissolved in 50 ml dry CH 2 Cl 2 again and cooled in an ice bath. A 10-ml CH 2 Cl 2 solution containing 15 mmol amine (1.5 equiv) and 20 mmol Et 3 N (2 equiv) was then added and the reaction mixture was stirred at room temperature under nitrogen atmosphere. After 1 h, the solution was treated with 50 ml water and 100 ml dichloromethane, and the organic phase was separated, dried, evaporated and then purified by column chromatography to form compound A with 90–95% yield. 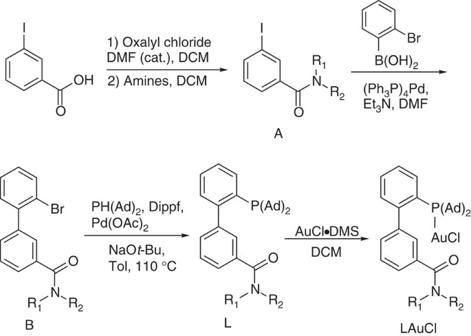Figure 6: Synthesis of ligands and catalysts. DCM, dichloromethane; DiPPF, bis(diisopropylphosphinyl)ferrocene; DMF,N,N-dimethylformamide; DMS, dimethylsulphide; Tol, toluene. Figure 6: Synthesis of ligands and catalysts. DCM, dichloromethane; DiPPF, bis(diisopropylphosphinyl)ferrocene; DMF, N , N -dimethylformamide; DMS, dimethylsulphide; Tol, toluene. Full size image A mixture of 8 mmol A (1 equiv), 8.8 mmol 2-bromophenylboronic acid (1.1 equiv) and 24 mmol Et 3 N (3 equiv) in 40 ml DMF was stirred and bubbled with N 2 gas for 15 min, and then 0.4 mmol Pd(PPh 3 ) 4 (5 mol %) was added; the reaction mixture was heated at 90 °C for 4–8 h under nitrogen atmosphere. Once thin layer chromatography (TLC) indicated that A was completely consumed, the reaction was diluted with 500 ml diethyl ether and washed with water to remove DMF. Then, the organic layer was dried over MgSO4, filtrated, evaporated and then purified by column chromatography to form product B with 85–92% yield. Under nitrogen atmosphere 2 mmol B (1 equiv), 0.1 mmol Pd(OAc) 2 (5 mol%), 0.12 mmol 1,1′-bis(diisopropylphosphino)ferrocene (6 mol%), 2.4 mmol sodium tert-butoxide (1.2 equiv) and 5 ml dry toluene were added to a flame-dried Schlenk flask and the resulting suspension was stirred until apparently homogenous (around 15 min). After adding 2.2 mmol di(1-adamantyl)phosphine (1.1 equiv), the flask was heated at 110 °C in oil bath for 12 h, which then was cooled to room temperature and purified by column chromatography without work-up to form final ligand L with 60–80% yield. To a suspension of 1 mmol ligand L in 5 ml anhydrous dichloromethane, chloro(dimethylsulphide)gold(I) (294.5 mg, 1 mmol) was added. The mixture was stirred for 30 min at room temperature and the solvent was evaporated off under reduced pressure to form the desired gold complex L AuCl in quantitative yield. For the detailed procedures and NMR and HRMS data, see Supplementary Methods . For the NMR and HRMS spectra of the ligands and catalysts, see Supplementary Figs 1–68 . General procedure for preparation of enol esters In a sealed 1 dr reaction vial equipped with a magnetic stirring bar, 3 mmol carboxylic acids (1 equiv), 4.4 mmol 1-hexyne (1.45 equiv) or 3.6 mmol other alkynes (1.2 equiv) and 3.1 mg NaBARF (1200, p.p.m.) were added to 0.6 ml fluorobenzene. L8AuNTf 2 (50 μl of a 3.09-mg ml −1 solution in PhF, 0.150 μmol, 50 p.p.m.) was added to the above vial and then the reaction mixture was heated at 80 °C for 12–24 h. Once TLC indicated the completion of the reaction, the reaction mixture was concentrated and left on the high vacuum pump for overnight to give the NMR-pure product. If crude NMR was not pure, the residue was further purified through silica gel flash chromatography to form the desired product. For the detailed procedures and NMR and HRMS data, see Supplementary Methods . For the NMR and HRMS spectra of the ligands and catalysts, see Supplementary Figs 69–158 . General procedure for one-pot sequence preparation of amides In a sealed 1 dr reaction vial equipped with a magnetic stirring bar, 3 mmol carboxylic acids (1 equiv), 4.4 mmol 1-hexyne (1.45 equiv) and 3.1 mg NaBARF (1200, p.p.m.) were added to 0.6 ml fluorobenzene. L8AuNTf 2 (50 μl of a 3.09-mg ml −1 solution in PhF, 0.150 μmol, 50 p.p.m. or 100 μl, 100 p.p.m.) was added to the above vial and then the reaction mixture was heated at 80 °C for 12–18 h. Once the reaction was completed using TLC, it was concentrated and left on the high vacuum pump for overnight to form the crude product, followed by adding 3.6 mmol amine (1.2 equiv) and stirring at 100 °C for 6–24 h. Once the reaction was completed by TLC, the mixture was purified through silica gel flash chromatography (eluents:ethyl acetate:hexanes=1:3) to form the desired product. For the detailed procedures and NMR and HRMS data, see Supplementary Methods . DFT calculation The details of the theoretical calculations are provided in the Supplementary Methods and Supplementary Data 1 . How to cite this article: Wang, Y. et al . A general ligand design for gold catalysis allowing ligand-directed anti-nucleophilic attack of alkynes. Nat. Commun. 5:3470 doi: 10.1038/ncomms4470 (2014). Accession codes: The X-ray crystallographic coordinates for structure L8AuCl reported in this article have been deposited at the Cambridge Crystallographic Data Centre (CCDC), under deposition number CCDC 985188. These data can be obtained free of charge from the Cambridge Crystallographic Data Centre via http://www.ccdc.cam.ac.uk/data_request/cif .